Mapping the oxygen structure of γ-Al2O3by high-field solid-state NMR spectroscopy γ-Al 2 O 3 is one of the most widely used catalysts or catalyst supports in numerous industrial catalytic processes. Understanding the structure of γ-Al 2 O 3 is essential to tuning its physicochemical property, which still remains a great challenge. We report a strategy for the observation and determination of oxygen structure of γ-Al 2 O 3 by using two-dimensional (2D) solid-state NMR spectroscopy at high field. 2D 17 O double-quantum single-quantum homonuclear correlation NMR experiment is conducted at an ultra-high magnetic field of 35.2 T to reveal the spatial proximities between different oxygen species from the bulk to surface. Furthermore, 2D proton-detected 1 H- 17 O heteronuclear correlation NMR experiments allow for a rapid identification and differentiation of surface hydroxyl groups and (sub-)surface oxygen species. Our experimental results demonstrate a non-random distribution of oxygen species in γ-Al 2 O 3 . Owing to their specific physical and chemical properties, metal oxides are of great importance in the field of materials and chemical science as diverse as electronics, energy storage and catalysis. In particular, the variability of their structure/phase and localized electronic structures has motivated widespread applications of metal oxides in heterogeneous catalysis [1] , [2] , [3] , [4] , [5] , [6] . γ-Al 2 O 3 is widely used in a broad range of industrial catalytic reactions such as alcohol dehydration, propane dehydrogenation, isomerization, alkylation and catalytic cracking [7] . Optimization and rational design of related heterogeneous catalysts rely on detailed knowledge of the structure–property relationship. Over the past decades, considerable efforts have been devoted to experimental and/or theoretical explorations of the structure and nature of γ-Al 2 O 3 , which however remain poorly understood [8] , [9] , [10] , [11] , [12] , [13] , [14] , [15] , [16] , [17] . Unambiguous determination of the location of Al and O atoms is hampered by the large line-broadening of reflections/diffuse scattering pattern of small γ-Al 2 O 3 particles in X-ray diffraction (XRD), neutron diffraction (ND) and electron diffraction characterizations. The surface species, particularly the coordinatively unsaturated atoms in γ-Al 2 O 3 are usually correlated with particle size, morphology and pretreatment conditions [18] , [19] , [20] . The oxygen speciation (e.g., hydroxyl or defects) of γ-Al 2 O 3 impacts its surface properties (i.e., acidity/basicity) , and in many cases the proposed catalytic mechanisms are closely related to the local environment of oxygen atoms [21] . Thus, determination of oxygen species in γ-Al 2 O 3 is prerequisite for understanding its structure and physicochemical property, which has remained a great challenge. Solid-state NMR spectroscopy is a powerful and versatile tool for structural characterization of materials in either ordered or disordered states via the measurement of nuclear spin interactions [22] , [23] , [24] , [25] , [26] . 17 O magic-angle spinning (MAS) NMR has been utilized in recent years to probe the local environments of oxygen atoms in various oxygen-containing materials [27] , [28] , [29] , [30] , [31] , [32] . However, a combination of quadrupolar nature for 17 O nucleus (I = 5/2), relatively low gyromagnetic ratio ( γ = −5.774 MHz T −1 ), and low 17 O abundance (0.037%) leads to great difficulties using 17 O NMR to investigate oxide-based materials especially at conventional magnetic fields (≤14.1 T). Therefore, the acquisition of 17 O MAS NMR spectrum often entails 17 O isotopic enrichment [33] . Additionally, advanced NMR methods and techniques are required to further enhance sensitivity and resolution. High-resolution two-dimensional (2D) experiments, such as 29 Si- 17 O heteronuclear correlation (HETCOR) and 17 O multiple-quantum (MQ) MAS experiments were reported in the structural characterization of inorganic materials (e.g., zeolite) [34] . Taking advantage of dynamic nuclear polarization (DNP) technique [35] , [36] , [37] , [38] , Pruski and coworkers showed the direct observation of Brønsted acid sites at natural abundance by 17 O DNP surface-enhanced NMR spectroscopy (SENS) on silica-alumina samples. Since continuous distribution of 17 O chemical shifts result in poor resolution of 17 O MAS NMR spectrum, the broad 17 O signals were analyzed by observing the change of their lineshapes associated with different hydroxyl environments (aluminols, silanols or Al(OH)Si) [39] . Our recent work showed that the surface oxygen sites with (e.g., aluminols and adsorbed water) or without (bare oxygen) bound protons on γ-Al 2 O 3 can be detected by 17 O DNP SENS through 2D 17 O MQMAS and 1 H- 17 O HETCOR experiments [40] . However, the determination of spatial proximity/connectivity between different oxygen sites has not been achieved yet, which is essential to better understand the local structure of γ-Al 2 O 3 . The conventional NMR approach is hampered by the small 17 O- 17 O interactions due to the low γ of the 17 O nucleus and the dilution from insufficient 17 O isotope enrichment. The oxygen speciation and its local structure in γ-Al 2 O 3 remain largely unknown. The emerging high magnetic field up to 35.2 T (1.5 GHz) with dramatically improved sensitivity and resolution opens new stage for the application of 17 O NMR spectrosopy [41] , [42] , [43] . In this contribution, we propose a strategy to unambiguously determine oxygen structure of γ-Al 2 O 3 with the aid of ultrahigh magnetic field and state-of-the-art pulse sequences. To the best of our knowledge, the 2D 17 O- 17 O double quantum (DQ)–single quantum (SQ) homonuclear correlation spectrum of γ-Al 2 O 3 is for the first time acquired at magnetic field of 35.2 T. Even for the γ-Al 2 O 3 sample with moderate 17 O labeling (ca. 20%), the 2D correlation maps can be achieved in several hours. 4-coordinated and 3-coordinated oxygen sites are identified and their spatial proximities between different oxygen species from the bulk to surface are revealed. In combination with 2D proton-detected 1 H- 17 O heteronuclear multiple quantum correlation (HMQC) experiments at 18.8 T, the discrimination of (sub-)surface oxygen species including bare oxygen, hydroxyl groups and adsorbed water is achieved. 3-coordinated oxygen sites are preferentially formed on the (sub-)surface of γ-Al 2 O 3 . Our 17 O NMR experimental results demonstrate a non-random distribution of oxygen species and a non-spinel structure in γ-Al 2 O 3 . The detailed insights into the oxygen sites provide a basis for tuning the property of γ-Al 2 O 3 and rational design of improved oxide-based catalysts. Identification of oxygen sites by 2D 17 O 3QMAS NMR Efficient enrichment of 17 O is essential for 17 O NMR spectroscopy especially the 2D correlation spectroscopy to study the structure of oxides. 17 O-enriched γ-Al 2 O 3 (BET surface area, 139.8 m 2 /g) was prepared with H 2 17 O (40%, 17 O) and boehmite. The labeled 17 O atoms in γ-Al 2 O 3 is less than 21% with respect to the total oxygen atoms in the sample (see Methods section for details). XRD and TEM image of the 17 O-enriched γ-Al 2 O 3 show the crystalline phase and morphology (see Supplementary Fig. 1 and Fig. 2 ). The IR data show the presence of different types of hydroxyl groups on γ-Al 2 O 3 (Supplementary Fig. 3 ), which are not influenced by 17 O isotope labeling treatment. The expected 4- and 6-coordinated Al (Al IV and Al VI ) sites along with a small amount of 5-coordinated Al (Al V ) on the sample are revealed by 27 Al MAS NMR (Supplementary Fig. 4a ). Raising dehydrated temperature from 473 to 673 K leads to a slight decrease of the Al VI accompanying with an increase of Al V (Supplementary Fig. 4a ). Therefore, the formation of Al V can be related to the dehydroxylation of surface Al VI , and a relatively higher treatment temperature would result in more Al V on the surface γ-Al 2 O 3 . It is noteworthy that there are many factors such as preparation method, morphology, particle size and post-treatment, could contribute to the variability of the surface property of γ-Al 2 O 3 [16] , [18] , [20] , [21] , [24] . The 17 O MAS NMR spectrum of 17 O labeled γ-Al 2 O 3 dehydrated at 473 K was acquired at 35.2 T. As shown in Fig. 1a , a main signal centered at ca. 71 ppm and high-field shoulders (ca. 50~65 ppm) are observed, which can be assigned to 4-coordinated (OAl 4 , denoted as O IV ) oxygen sites and 3-coordinated (OAl 3 , denoted as O III ) oxygen sites [15] , [44] , respectively. The high-field signals at ca. −10~40 ppm are resolved as well, which are broadened and indistinguishable at lower magnetic field of 18.8 T due to the low concentration and quadrupolar broadening (Supplementary Fig. 4b ). These weak signals can be assigned to the surface hydroxyl groups [40] . In order to make a clear determination of these oxygen species, 2D triple-quantum (3Q) MAS experiments were conducted at 35.2 T and 18.8 T, respectively (Fig. 1b, c ). The two overlapped resonances from the O IV (O(Al) 4 ) and O III (O(Al) 3 ) sites in the 1D 17 O MAS NMR spectrum become well resolved in the 2D 3QMAS spectra, which allows for assignment of different types of oxygen species by their chemical shifts. The distribution of chemical shift rather than the quadrupolar broadening dominates the lineshape of the 17 O NMR spectrum at high field of 35.2 T, hence it enables to deconvolute the isotropic projection of the 2D 17 O 3QMAS by using five individual Gaussian lines (sites A-E in Fig. 1b ). Sites B, C and D can be easily identified, while A and E are not well discriminable owing to their low concentrations. To further probe these oxygen sites, 2D 17 O 3QMAS spectrum was also recorded at lower field of 18.8 T, in which the quadrupolar interactions of different oxygen sites could lead to discontinuous evolution of the chemical shift distribution (Fig. 1c ). Besides sites B, C and D, sites A and E become well resolved by the cross-sections in the 2D spectrum. The existence of oxygen A and E is further confirmed by the following 2D 17 O DQ-SQ homonuclear correlation and 1 H { 17 O} HMQC experiments (see the next sections). The 3QMAS experiment does not provide significant spectral resolution, which can be account for by the facts including relatively small quadrapolar coupling constant ( C Q ), very high magnetic field ( B 0 ) and broad chemical shift distribution for multiple sites in γ-Al 2 O 3 . Nevertheless, the deviation from the line with C Q = 0 (the green line in Fig. 1b, c ) reflect how large the quadrupole shift is and allow for more precise determination of the chemical shift by subtracting or taking the quadrupole shift into account. 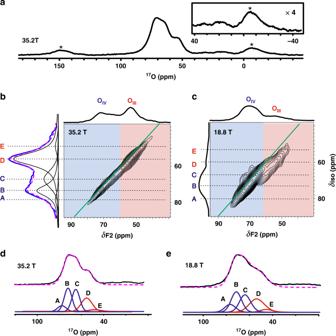Fig. 1: Identification of oxygen sites by 1D17O MAS NMR and 2D17O 3QMAS NMR. a1D17O MAS NMR spectrum of γ-Al2O3acquired at 35.2 T and partially enlarged17O spectrum,bsheared 2D17O 3QMAS spectrum of γ-Al2O3recorded on 35.2 T and projection (blue) in isotropic dimension with the simulated spectrum (purple) deconvoluted by five individual Gaussian lines (black, A-E denote as five individual oxygen sites),csheared 2D17O 3QMAS spectrum of γ-Al2O3recorded at 18.8 T. Green lines in 2D spectra represent chemical shift/diagonal axis (CQ= 0). OIVand OIIIdenote 4-coordinated and 3-coordinated oxygen sites, respectively.d,eThe best-fit simulation spectra (purple) of the 1D17O MAS NMR spectra (black) of γ-Al2O3obtained at 35.2 T and 18.8 T. The 1D spectra are deconvoluted with the DMFIT program57according to the NMR parameters of five oxygen sites (A-E) in TableS1. The acquisition times of the 2D17O 3QMAS spectra at 35.2 T and 18.8 T are ca. 0.53 h and ca. 40 h, respectively. Asterisks denote spinning sidebands. Supplementary Table 1 lists the NMR parameters of all the oxygen species extracted from the 2D 17 O 3QMAS spectra at two fields. Accordingly, the 1D 17 O MAS NMR spectra obtained at the two fields can be well fitted by the five oxygen sites (Fig. 1d, e ). Fig. 1: Identification of oxygen sites by 1D 17 O MAS NMR and 2D 17 O 3QMAS NMR. a 1D 17 O MAS NMR spectrum of γ-Al 2 O 3 acquired at 35.2 T and partially enlarged 17 O spectrum, b sheared 2D 17 O 3QMAS spectrum of γ-Al 2 O 3 recorded on 35.2 T and projection (blue) in isotropic dimension with the simulated spectrum (purple) deconvoluted by five individual Gaussian lines (black, A-E denote as five individual oxygen sites), c sheared 2D 17 O 3QMAS spectrum of γ-Al 2 O 3 recorded at 18.8 T. Green lines in 2D spectra represent chemical shift/diagonal axis ( C Q = 0). O IV and O III denote 4-coordinated and 3-coordinated oxygen sites, respectively. d , e The best-fit simulation spectra (purple) of the 1D 17 O MAS NMR spectra (black) of γ-Al 2 O 3 obtained at 35.2 T and 18.8 T. The 1D spectra are deconvoluted with the DMFIT program [57] according to the NMR parameters of five oxygen sites (A-E) in Table S1 . The acquisition times of the 2D 17 O 3QMAS spectra at 35.2 T and 18.8 T are ca. 0.53 h and ca. 40 h, respectively. Asterisks denote spinning sidebands. Full size image Distortions in the geometry of O(Al) n ( n = 3–4) sites lead to the variations for P Q (quadrupole interaction product) and δ cs (isotropic chemical shift) values (see Supplementary Table 1 ), as observed in the case of γ-alumina [15] , glasses [45] and zeolites [34] . In comparison, O III sites D-E exhibit larger quadrupolar couplings (2.7–3.1 MHz) than that of O IV sites A-C (1.8–2.4 MHz). This can be understood by the fact that O III sites experience larger distortions of local environment induced by cation vacancies or surface defects in γ-Al 2 O 3. Since the high-field signals (ca. −10–40 ppm) from hydroxyl groups are too weak to be observed in the 2D 3QMAS spectra, all these resolved signals come from the oxygen species without bound protons. Determination of oxygen-oxygen structures by 2D 17 O DQ-SQ experiment Up to now, there is no report yet on detecting the spatial proximity/connectivity of oxygen species in γ-Al 2 O 3 largely due to insufficient 17 O enrichment, detection sensitivity and spectral resolution required to correlate two low-γ S = 5/2 spins. For a specific nucleus, high magnetic fields lead to increase of its Larmor frequency and the net magnetization from the population difference between the neighboring energy levels (e.g., 1/2 ↔ −1/2), thus enhancing NMR signal through both resonance frequency and the polarization. More importantly for quadrupole nuclei, high fields reduce the broadening from the second-order quadrupolar effect, therefore provide a gain of spectral resolution proportional to the square of B 0 in units of ppm [46] . With the aid of our developed BR2 1 2 pulse sequence [47] and the dramatic sensitivity and resolution enhancement achieved by the Series-Connected Hybrid magnet capable of generating magnetic field of up to 35.2 T [42] , 2D 17 O DQ-SQ homonuclear correlation spectrum was obtained on γ-Al 2 O 3 sample in less than 4 h (Fig. 2a ). Despite a low radio-frequency recoupling field (ca. 2.7 kHz) was used in the 2D 17 O DQ-SQ NMR experiment, our previous work [47] has demonstrated that the BR2 1 2 recoupling employed here was sufficient to cover a bandwidth of ca. 8 kHz (i.e., 45 ppm–80 ppm at 35.2 T). To the best of our knowledge, this is the first report of the 2D 17 O DQ-SQ homonuclear correlation spectrum, which provides a direct view of the dipolar interactions between different types of oxygen species and thus of their spatial proximity. Fig. 2: Probing oxygen-oxygen proximities via 2D 17 O double quantum (DQ)- single quantum (SQ) experiments. a 2D 17 O MAS DQ-SQ homonuclear correlation NMR spectrum of γ-Al 2 O 3 recorded at 35.2 T and b extracted slices along F2 dimension. The acquisition time for the 2D spectrum is ca. 3.7 h. O IV and O III denote 4-coordinated and 3-coordinated oxygen sites, respectively. A-E denote five individual oxygen sites, A-A, B-B, C-C and D-D represent the auto-correlations from the same oxygen sites, B-E, C-D and B-D represent the cross-correlations from two distinct oxygen sites. The purple arrows in b indicate the position of two coupled oxygen sites in the extracted slices. Full size image Since the dipolar interaction is inversely proportional to the cube of the distance between two 17 O atoms, the detected correlations in Fig. 2a should mainly originate from 2-bond 17 O-Al- 17 O correlation rather than 4-bond 17 O-Al-O-Al- 17 O correlation by considering the transfer efficiency as well as the dipolar truncation effect of the homonuclear recoupling [48] . Moreover, simulations were performed to compare DQ-SQ experimental efficiencies between isolated 2-bond and 4-bond 17 O pair (Supplementary Fig. 5 ) based on the non-spinel γ-Al 2 O 3 model [11] . The simulated double-quantum filtering (DQF) efficiency of the former remains over ten times higher than that of the latter at the point of experimental DQ recoupling time ( τ re = 3 ms) although the dipolar truncation effect is not taken into account. This suggests the detected correlations in Fig. 2a should mainly originate from 2-bond 17 O-Al- 17 O correlation. Four self-correlation peaks (A-A, B-B, C-C, and D-D) are observed along the diagonal line with a slope of 2, indicating the same types of the oxygen sites are in close proximity one another. 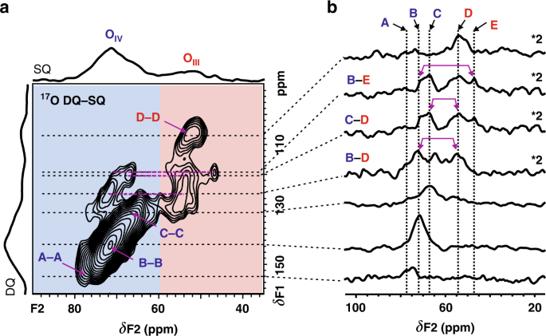Fig. 2: Probing oxygen-oxygen proximities via 2D17O double quantum (DQ)- single quantum (SQ) experiments. a2D17O MAS DQ-SQ homonuclear correlation NMR spectrum of γ-Al2O3recorded at 35.2 T andbextracted slices along F2 dimension. The acquisition time for the 2D spectrum is ca. 3.7 h. OIVand OIIIdenote 4-coordinated and 3-coordinated oxygen sites, respectively. A-E denote five individual oxygen sites, A-A, B-B, C-C and D-D represent the auto-correlations from the same oxygen sites, B-E, C-D and B-D represent the cross-correlations from two distinct oxygen sites. The purple arrows inbindicate the position of two coupled oxygen sites in the extracted slices. While the cross peaks B-E, C-D and B-D reflect the spatial proximities between different oxygen species, which could be unambiguously identified in the 1D slices extracted from the 2D spectrum (Fig. 2b ). Although the correlation peaks mainly depend on the strength of dipolar coupling (O-Al-O distance), the concentration of the proximate oxygen pairs contribute to the relative intensities as well. As shown in the 1D 17 O MAS spectrum (Fig. 1 ) and 2D 17 O DQ-SQ NMR spectrum (Fig. 2a ), the signal B is more intense than the others. Thus, site B is most likely present as bulk species in γ-Al 2 O 3 . This is further supported by the fact that site B correlates with the other high-field O III sites (D and E) (Fig. 2b ). For the O III site D, there is a downfield shift (1~2 ppm) of the center of gravity in its cross peaks (e.g., B-D) compared with its self-correlation peak (D-D). This implies that the slight difference of the oxygen-oxygen local structure in γ-Al 2 O 3 might be an important factor influencing the distribution of electric field gradients (EFG) of oxygen sites, which yields a distribution of apparent chemical shifts of 17 O NMR involving the isotropic quadrupolar shift. Note that an off-diagonal signal (ca. 78 ppm in F2 dimension) at the lowest field seriously overlaps with self-correlation peaks A-A and B-B. This off-diagonal correlation could be either the correlation between two A sites with continuous chemical shift distributions caused by slightly different local environments or the cross correlation between A and B. No additional cross-peak is observable with respect to site A, indicating that either this type of oxygen is not located in close proximity to other oxygen sites or there are less proximate oxygen pairs between site A and other oxygen sites. In addition, there is no apparent cross correlation between two distinct O IV species (e.g., B-C, A-C) in the 2D 17 O DQ-SQ spectrum (Fig. 2a ), which suggests that different magnetically inequivalent O IV sites are separated. Similarly, no cross correlation between site D and E observed in Fig. 2a reveals that these two O III species are not in close proximity. These experimental results suggest that different oxygen species (magnetically inequivalent) discriminated here are closely related to their special O-Al-O local structures. Taking the information obtained from the 2D DQ-SQ NMR experiment together, it provides the first direct evidence that these oxygen sites in γ-Al 2 O 3 exist in a non-random manner. Discrimination of surface oxygen species by 2D 1 H{ 17 O} HMQC experiment Note that it’s not straightforward to correlate the surface oxygen species with that in the bulk by above 17 O 3QMAS and DQ-SQ experiments since the surface oxygen species that are in form of hydroxyl groups are not observed in the 2D NMR spectra (Figs. 1 and 2 ). 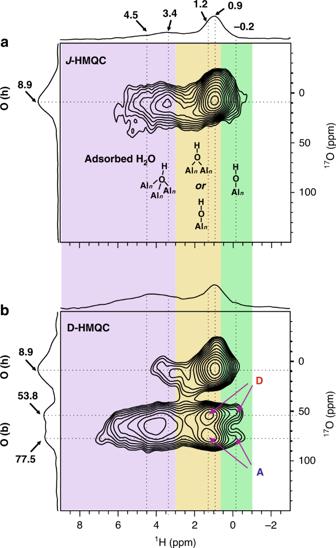Fig. 3: Discrimination of surface oxygen species by 2D1H{17O} HMQC experiments. a2D1H{17O}J-HMQC spectrum andb2D1H{17O} D-HMQC spectrum of γ-Al2O3withτre= 1.05 ms recorded at 18.8 T. The background colors differentiate the hydroxyl groups based on their isotopic chemical shifts in the1H dimension. The oxygen species associated with hydroxyls and the bare oxygen species are denoted as O(h) and O(b), respectively. The structure of triply bridging, doubly bridging and terminal hydroxyls are displayed in Fig.3abased on the distribution of respective1H chemical shifts. A and D indicate the specific 4-coordinated and 3-coordinated oxygen sites, respectively, which are correlated with doubly bridging and terminal hydroxyls in Fig.3b. The acquisition time for theJ- and D-HMQC spectra is ca. 4.6 and 9.1 h, respectively. By taking advantage of localized interactions between protons and oxygen, 1 H- 17 O HETCOR experiment could provide selective information on the surface hydroxyl groups and even the surface bare oxygen species provided the proton source such as hydroxyl group or adsorbed water are in close proximity to the target oxygen sites. However, the use of conventional 1 H- 17 O cross polarization (CP) or 17 O{ 1 H} D-HMQC NMR experiment is time-consuming for quadrupolar nucleus with low γ and at low natural abundance [49] , [50] . Owing to the high sensitivity of 1 H nuclei, proton-detected HETCOR experiments such as HMQC [51] , R-INEPT [32] and TEDOR [43] have proved to be robust methods to indirectly detect the insensitive nuclear spin as well as to explore its connectivity/proximity with proton under fast MAS. Since a single-resonance 3.2 mm probe was equipped on the 35.2 T NMR system which could not render fast MAS and double-resonance experiment, Therefore, we conducted the proton-detected 2D 1 H { 17 O} J /D-HMQC experiments using a 1.9 mm double-resonance probe on a commercial at 18.8 T NMR spectrometer with a MAS speed of 40 kHz. The 1 H- 17 O J -HMQC through-bond experiment allows for identification of hydroxyl groups (-OH) exposed on γ-Al 2 O 3 , while the 2D 1 H- 17 O D-HMQC through-space experiment was used to probe bare oxygen (without H bonded) in close proximity with hydroxyl groups. The through-space method enables to detect bare 17 O not only on the surface but also below the surface (denoted as sub-surface) provided there are similar internuclear distances (or dipolar interactions) between these bare oxygens and protons of surface hydroxyls. According to previous experimental and theoretical reports [16] , [39] , the O-H bond length on γ-Al 2 O 3 is about 1 Å with the corresponding J coupling of ca. 80 Hz. The 2D proton-detected 1 H { 17 O} J- HMQC spectrum in Fig. 3a shows the chemical bond correlations through scalar-coupling transfer in which only the 1 H- 17 O correlations from hydroxyl groups are observable. Although the 17 O signals from different hydroxyl groups are severely overlapped in the 17 O dimension, the distinguishable 1 H signals help assign the hydroxyl groups on the surface of γ-Al 2 O 3 . The surface hydroxyl groups have been extensively examined by 1 H solid-state NMR spectroscopy [18] , [20] , [24] , [52] . Three main spectral regions were identified at around 0 ppm, 1-3 ppm and 3-5 ppm, which fall into the chemical shift range of terminal (μ 1 ) hydroxyl, doubly bridging (μ 2 ) hydroxyl and triply bridging (μ 3 ) hydroxyl groups, respectively. While the very recent work by Raybaud [20] indicated that besides the exposed main surface of γ-Al 2 O 3 , the stepped surfaces and edges architectures should be taken into account to interpret the 1 H NMR as well. Specifically, the −0.2 ppm 1 H signal comes from the μ 1 -OH; the proton 0.9 and 1.2 ppm signals can be assigned to the μ 2 -OH or μ 1 -OH, while the signal at 3.4 ppm is ascribed to the μ 3 -OH. Besides, chemically adsorbed H 2 17 O is observed on the sample surface reflected by the broad correlations at 1 H chemical shift larger than 4.0 ppm, which is confirmed by the dramatic decrease of the corresponding 1 H signal on the sample when dehydration temperature is raised from 473 K to 673 K (Supplementary Fig. 4c ). The 2D 1 H{ 17 O} J -HMQC experiment directly reveals different types of hydroxyl groups through directly connecting oxygen with proton atoms. These surface hydroxyl groups confirm the observation of the weak high-field 17 O signals in the 17 O MAS NMR spectrum (Fig. 1a ). Compared with the 1D 1 H MAS NMR spectrum, a significant decline in the 1 H signals (ca. 4.5 ppm) from adsorbed H 2 O is observed in the 2D 1 H{ 17 O} J -HMQC, implying much faster transverse relaxation of protons in the residual water molecules than that in hydroxyl groups on the surface of γ-Al 2 O 3 . Meanwhile the stronger intensity of the correlation peak in the 2D spectrum suggests that the μ 2 -OH dominates the surface hydroxyl groups on our γ-Al 2 O 3 samples. Fig. 3: Discrimination of surface oxygen species by 2D 1 H{ 17 O} HMQC experiments. a 2D 1 H{ 17 O} J -HMQC spectrum and b 2D 1 H{ 17 O} D-HMQC spectrum of γ-Al 2 O 3 with τ re = 1.05 ms recorded at 18.8 T. The background colors differentiate the hydroxyl groups based on their isotopic chemical shifts in the 1 H dimension. The oxygen species associated with hydroxyls and the bare oxygen species are denoted as O(h) and O(b), respectively. The structure of triply bridging, doubly bridging and terminal hydroxyls are displayed in Fig. 3a based on the distribution of respective 1 H chemical shifts. A and D indicate the specific 4-coordinated and 3-coordinated oxygen sites, respectively, which are correlated with doubly bridging and terminal hydroxyls in Fig. 3b . The acquisition time for the J - and D-HMQC spectra is ca. 4.6 and 9.1 h, respectively. Full size image The 1 H{ 17 O} J -HMQC spectrum shows detailed information about chemical connectivity between surface oxygen and protons. In order to get extended picture of the surface oxygen structure, 2D 1 H{ 17 O} D-HMQC experiments were also conducted on γ-Al 2 O 3 . The 1 H{ 17 O} D-HMQC experiment uses the dipolar interaction to create correlation signal, which is more robust than the commonly used CP/MAS sequence for the investigation of spatial proximity between quadrupolar and spin-1/2 nuclei [53] . The variation of the recoupling time allows to probe local environment of the surface oxygen at various distances to hydroxyl protons. The 1 H{ 17 O} D-HMQC spectrum of γ-Al 2 O 3 with a short recoupling time of 0.30 ms shows correlations to the neighboring species at short distance (Supplementary Fig. 6 ), similar to those achieved by the J -based experiment. Increasing the recoupling time to 1.05 ms gives rise to additional signals in Fig. 3b . Besides the 1 H- 17 O correlations from different bridging hydroxyl groups ( 17 O chemical shift at ca. −10–40 ppm), strong correlations between the protons of hydroxyl groups and the 17 O signals at ca. 50–75 ppm are observed. The well-resolved low-field 17 O signals can be assigned to oxygen site A and D, respectively, by considering their apparent 17 O chemical shifts ( δ F2 ). 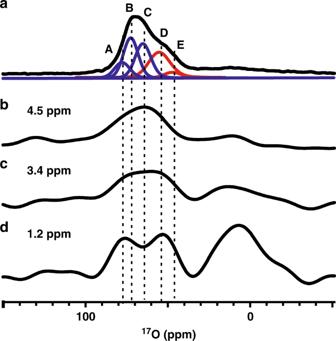Fig. 4: Comparison of specific17O NMR slices extracted from Fig.3b. Deconvolution lines of 1D17O MAS NMR spectrum at 18.8 T (a), and extracted17O NMR slices from 4.5 ppm (b), 3.4 ppm (c) and 1.2 ppm (d) in the1H dimension of 2D1H{17O} D-HMQC spectrum (Fig.3b), respectively. Letters A-C denote three fitted 4-coordinated oxygen sites (blue lines), D-E denote two fitted 3-coordinated oxygen sites (red lines). 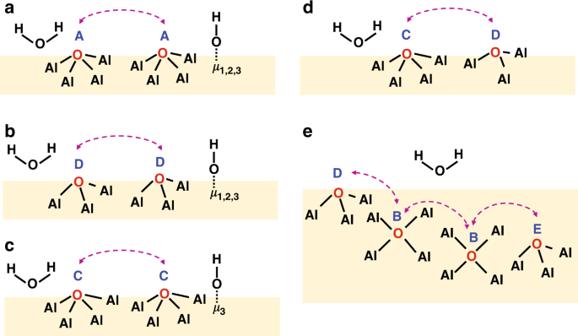Fig. 5: Proposed local structure models of oxygen species in γ-Al2O3. a–eLetters A-E represent five distinct bare oxygen sites. The purple dotted arrows indicate the spatial proximities between two specific bare oxygen sites. Surface terminal (μ1), doubly (μ2) and triply (μ3) bridging hydroxyl groups are indicated. Figure 4 displays the selective 1D slice of the 17 O NMR spectra along different 1 H chemical shifts (1.2 ppm, 3.4 ppm and 4.5 ppm) extracted from the 2D 1 H- 17 O D-HMQC spectrum. The correlation peaks indicate that the μ 1 -OH and μ 2 -OH groups (−0.2–2.0 ppm) are mainly located in close proximity to O IV site A and O III site D (also see Fig. 4d ). Although it is difficult to differentiate 17 O sites from the 1D 17 O slices along the 1 H signals at 3.4 ppm (Fig. 4c ) and 4.5 ppm (Fig. 4b ), the lineshape of the 17 O slice for the latter implies that water molecule (4.5 ppm) is preferentially adsorbed on O IV site C, showing its strong hydrophilicity on the surface of γ-Al 2 O 3 . While the intramolecular 1 H- 17 O correlations for chemically adsorbed H 2 17 O are hard to be observed, which can be accounted for by the relatively faster relaxation of the nuclear spins in water molecule during the period of dipolar recoupling. Note that different 1 H species have distinct influences on the intensities of 1 H- 17 O correlations in 2D HMQC experiment due to their different relaxations. We analyzed the 1 H- 17 O correlation slices extracted from specific 1 H resonances (i.e., 4.5 ppm, 3.4 ppm and 1.2 ppm in 1 H dimension, see Fig. 4 ). For a specific 1 H resonance, its transverse relaxation would attenuate its 1 H- 17 O correlations on similar level in 2D HMQC spectra, which would thus does not significantly influence the relative intensities of distinct 17 O species in its 1 H- 17 O correlation slice in the 17 O dimension. Fig. 4: Comparison of specific 17 O NMR slices extracted from Fig. 3b . Deconvolution lines of 1D 17 O MAS NMR spectrum at 18.8 T ( a ), and extracted 17 O NMR slices from 4.5 ppm ( b ), 3.4 ppm ( c ) and 1.2 ppm ( d ) in the 1 H dimension of 2D 1 H{ 17 O} D-HMQC spectrum (Fig. 3b ), respectively. Letters A-C denote three fitted 4-coordinated oxygen sites (blue lines), D-E denote two fitted 3-coordinated oxygen sites (red lines). Full size image No apparent correlations are observed between protons and oxygen site B in the 2D D-HMQC spectrum. This is a clear indication that this oxygen species should be not in close proximity to the surface protons. The longer internuclear distance makes the dipolar interaction too weak to be detected by the D-HMQC experiment. Taking the results together, it strongly suggests that site B exist in the bulk while sites A, C and D are most likely present on the (sub-)surface of γ-Al 2 O 3 . The influence of the heating treatment on the distribution of the surface oxygen species on γ-Al 2 O 3 was analyzed by 1 H{ 17 O} D-HMQC. 17 O MAS NMR (Supplementary Fig. 4b ) shows that there is an apparent decrease of the 17 O signals from the hydroxyl groups (ca. −10–45 ppm) along with the increase of the 17 O signals from bare oxygen species (ca. 45–80 ppm) on γ-Al 2 O 3 when the dehydration temperature is raised from 473 to 673 K. Interestingly, the 1 H- 17 O correlations revealed by the 2D 1 H{ 17 O} D-HMQC spectrum of γ-Al 2 O 3 dehydrated at 673 K (Supplementary Fig. 7 ) are quite similar to those observed on the sample dehydrated at lower temperature (Fig. 3b ). In particular, the residual μ 2 -OH and μ 1 -OH (−0.2–2.0 ppm) on γ-Al 2 O 3 keep close proximity to the specific O IV (e.g., site A) and O III (e.g., site D) species. This indicates that heating treatment at mild condition does not have significant impact on the structure of the surface oxygen species on γ-Al 2 O 3 . The detailed information about the oxygen speciation and spatial proximities and connectivities of different oxygen sites allows us to propose local structure models of γ-Al 2 O 3 (Fig. 5 ). The (sub-)surface of γ-Al 2 O 3 is occupied by different types of oxygen sites (A, C and D) which are in close proximity to surface hydroxyl group or water molecule (Fig. 5a–c ). The O IV (site C) and O III (site D) species are found to be located in close proximity as well (Fig. 5d ). In spite of the low concentration, oxygen site E that is mostly likely in the bulk can still be identified based on its spatial proximity with oxygen site B (Fig. 5e ). While the bulk oxygen site B is probably located near to the surface of γ-Al 2 O 3 as evidenced by its proximity to site D. Fig. 5: Proposed local structure models of oxygen species in γ-Al 2 O 3 . a – e Letters A-E represent five distinct bare oxygen sites. The purple dotted arrows indicate the spatial proximities between two specific bare oxygen sites. Surface terminal (μ 1 ), doubly (μ 2 ) and triply (μ 3 ) bridging hydroxyl groups are indicated. Full size image The complex oxygen species in γ-Al 2 O 3 in terms of speciation and distribution often bring about difficulty in the characterization of their structures and properties. This is demonstrated by the overlapping 17 O signals and insufficient spectral resolution even in the 2D 17 O 3QMAS spectrum recorded at high field (Fig. 1b, c ). The high-resolution cross peaks provided by the 2D 17 O DQ-SQ and 1 H { 17 O} HMQC spectra enables to resolve and determine these overlapped components. This makes the quantitative measurements of distinct oxygen species feasible on the 1D 17 O NMR spectra (Fig. 1d, e ). The 17 O NMR spectra allow to not only obtain unprecedented information on the local environment of oxygen species but also shed insight into the structure of γ-Al 2 O 3 by analyzing the location of Al 3+ vacancies [17] . In the spinel-like model, the vacancy at an octahedral position results in the formation of six O III anions. While the vacancy at a tetrahedral position produces four O III anions, leading to a non-spinel structure [11] . Therefore, the γ-Al 2 O 3 bulk structure could be determined via a quantitative analysis of O IV and O III sites in 1D 17 O MAS NMR spectrum. For example, the O III /O IV ratio in a unit cell of Al 8 O 12 is 1.0 or 0.5 for an Al 3+ vacancy at octahedral or tetrahedral position, respectively. The deconvolutions of 1D 17 O MAS NMR spectra of γ-Al 2 O 3 (Fig. 1d, e ) assisted by the improved resolution of the 2D 17 O DQ-SQ and 1 H { 17 O} D-HMQC spectra clearly show an O III /O IV ratio of 0.51 ± 0.03 at 18. 8 T or 0.45 ± 0.04 at 35.2 T (Supplementary Table 1 ), respectively, suggesting that Al vacancies should be located at tetrahedral position. In addition, 27 Al MAS NMR spectroscopy allows for the determination of the location of the Al vacancies in γ-Al 2 O 3 by measuring the proportion of octahedral Al VI or tetrahedral Al IV sites. If the vacancies (V) are at octahedral positions, γ-Al 2 O 3 is expressed as Al IV [Al 5/3 V 1/3 ] VI O 4 and 62.5% Al 3+ cations are located at octahedral positions [17] . For the vacancies at tetrahedral positions, γ-Al 2 O 3 gives a the formula of [Al 2/3 V 1/3 ] IV [Al 2 ] VI O 4 and there are 75% Al 3+ cations at octahedral positions. The 1D 27 Al MAS spectrum of γ-Al 2 O 3 dehydrated at 473 K (Supplementary Fig. 4a ) shows that 73% of Al 3+ cations is in octahedral coordination, confirming that the vacancies are mainly at tetrahedral positions. This is also in agreement with previous 27 Al DQ-SQ experimental result on γ-Al 2 O 3 [54] , where there is no correlation from two coupled tetrahedral 27 Al observed in the 2D 27 Al homonuclear correlation spectrum. It should be noted that the thermal treatment impacts to some extent the coordination of Al atom in γ-Al 2 O 3 . As shown in Supplementary Fig. 4a , the 6-coordinated Al decreases from 73% to 70% upon increasing the dehydration temperature from 473 to 673 K. Note that there is a small variation (from 67.5% to 75%) of Al VI upon varying vacancies from octahedral to tetrahedral Al. This would lead to a larger measurement error on the amount of vacancies at tetrahedral or octahedral positions in 27 Al MAS NMR compared with that obtained in 1D quantitative 17 O MAS NMR. Nevertheless, the Al vacancies are predominately located at tetrahedral positions, which is a clear indication of the non-spinel structure for γ-Al 2 O 3 . In our previous DNP study of γ-Al 2 O 3 [40] , surface-selectively labeling was performed by surface exchange of commercial γ-Al 2 O 3 with 17 O 2 gas or H 2 17 O. In addition to the surface hydroxyl groups, O III and O IV species were observed. Aiming at a detailed understanding of oxygen species in γ-Al 2 O 3 , herein we investigated the labeled samples both on the surface and in the bulk which were prepared by dehydration of 17 O-enriched boehmite. The thermal treatment would influence more or less the oxygen species particularly on the surface of γ-Al 2 O 3 . For example, the surface hydroxyl groups were obviously decreased with increasing of dehydration temperature, which was confirmed by our 1D 17 O and 1 H MAS NMR spectra (Supplementary Fig. 4b and 4c ). In spite of the variation of surface species, the 2D 1 H- 17 O D-HMQC spectrum revealed the preferential formation of O III species on the (sub-)surface of γ-Al 2 O 3 (Fig. 3b ), in agreement with the result obtained by the direct 17 O DNP spectroscopy [40] . The basic property of γ-Al 2 O 3 is related to surface oxygen sites. For example, the terminal surface hydroxyl group was found to have selective reactivity toward CO 2 [24] . Some active sites (so called defect sites) are supposed to be formed by the Lewis acid (tri-coordinated Al)–base (O) pairs on the metastable surface of γ-Al 2 O 3 [21] . Furthermore, the surface oxygen on γ-Al 2 O 3 could serve as the anchoring site for metal supported catalysts. The distribution of the (sub-)surface oxygen especially the coordinately unsaturated oxygen such as site D led us to believe that the anchoring of the supported metal species on γ-Al 2 O 3 would be non-random. The isolated or vicinal oxygen sites would influence the formation of metal ions or clusters, which have been demonstrated to exhibit distinct activity [55] . In summary, we provide a robust and reliable 17 O NMR strategy to map the oxygen structure in γ-Al 2 O 3 . The combined high magnetic fields and fast MAS demonstrate the ability to increase the sensitivity and resolution of 2D 17 O MAS NMR spectra. Different oxygen species and their spatial proximities in γ-Al 2 O are identified by 17 O 3QMAS in combination of 2D 17 O DQ-SQ homonuclear correlation NMR experiments conducted at 35.2 T. The proton-detected 1 H- 17 O J /D-HMQC experiments allow a rapid detection of the (sub-)surface oxygen species through chemical bond or spatial/dipolar interaction with surface protons including water and hydroxyl groups. The results presented herein not only provide unique insights into the structure of oxygen sites of γ-Al 2 O 3 , which has important implications for tuning the property of γ-Al 2 O 3 , but also demonstrate the ability to utilize the increased resolution/sensitivity of 2D 17 O NMR experiments at high or ultra-high magnetic fields to investigate various complex metal oxide-based catalysts. The detailed information on oxygen speciation and its local structure would enable to better understand the anchoring site for supporting metals as well as the specific interaction between oxides surface and reaction molecules, which is helpful for the rational design of improved catalysts. Preparation of 17 O enriched γ-Al 2 O 3 17 O-enriched boehmite was first prepared by exchanging boehmite with H 2 17 O. 380 μl (0.38 g) H 2 17 O ( 17 O, 40%) was introduced into a glass tube containing 500 mg pretreated AlOOH•H 2 O. The glass tube was sealed with a flame after degassing on a vacuum line at 423 K for 48 h. Then, 17 O-enriched γ-Al 2 O 3 was prepared by dehydration of the 17 O-enriched boehmite at 773 K for 4 h. Consequently, the enriched γ-Al 2 O 3 samples were dehydrated at 473 K or 673 K for 2 h and were stored in sealed glass tube to minimize adsorption of atmospheric moisture. The amount of 17 O labeling can be roughly estimated. A total of~ 20 mmol of H 2 17 O ( 17 O, 40%) was used for 500 mg of AlOOH•H 2 O. The maximum labeled 17 O atoms should be less than 21% ([20 mmol*40%( 17 O)]/[20 mmol( \({\rm{O}}_{{\rm{H}}_{2}{\rm{O}}} \) ) + 19.5 mmol( \({\rm{O}}_{{\rm{AlOOH•}} {{\rm{H}}_{2}{\rm{O}}}} \) )]) with respect to the total oxygen atoms of the sample. Solid-state NMR measurements 1D 17 O MAS NMR, 2D 17 O 3QMAS and DQ-SQ MAS NMR spectra were recorded on 35.2 T series-connected hybrid magnet at the National High Magnetic Field Laboratory (NHMFL) using a Bruker Avance NEO console and a single-resonance 3.2 mm MAS probe designed and constructed at the NHMFL. A pulse width of 3 µs corresponding to a π/6 flip-angle and a recycle delay of 1 s were used to collect the single-pulse 17 O MAS NMR spectrum of γ-Al 2 O 3 at a spinning speed of 15.6 kHz. The number of transients collected was 128. The 2D 17 O 3QMAS spectrum of γ-Al 2 O 3 was collected using a shifted-echo sequence, and all pulse widths were optimized on the sample at a spinning speed of 15 kHz. A total of 48 scans were collected for each of the 40 rotor-synchronized t 1 increments with a recycle delay of 1 s. 2D 17 O DQ-SQ MAS NMR experiment was conducted using BR2 1 2 recouplings ( τ re = 3 ms), and all pulse widths were optimized at a spinning speed of 16 kHz. Central transition (CT) enhancement of the initial magnetizations ( 17 O) was obtained by using a SS-WURST-80 irradiation with a length of 1 ms. A total of 832 scans were collected for each of the 16 rotor-synchronized t 1 increments with a recycle delay of 1 s. 1D 17 O MAS NMR and 2D 17 O 3QMAS spectra were also recorded on 18.8 T with a MAS speed of 15 kHz by using a Bruker Avance III 800 spectrometer and a 3.2 mm double resonance probe. A pulse width of 1.3 µs corresponding to a π/6 flip-angle and a recycle delay of 0.5 s were used to collect the single-pulse 17 O MAS NMR spectrum with 1600 scans. The 2D 17 O 3QMAS spectrum of γ-Al 2 O 3 was collected using a z-filtering sequence, and all pulse widths were optimized on the sample at a spinning speed of 15 kHz. A total of 2400 scans were collected for each of the 40 t 1 increments (Δ t 1 = 50 μs) with a recycle delay of 1.5 s. 1D single-pulse 27 Al, 1 H and 17 O MAS NMR spectra were collected at 18.8 T with a MAS speed of 40 kHz by using a 1.9 m double-resonance probe. A pulse width of 1.85 µs corresponding to a π/2 flip-angle and a recycle delay of 10 s were used to collect the single-pulse 1 H MAS NMR spectrum with 8 scans. A pulse width of 0.7 µs corresponding to a π/6 flip-angle and a recycle delay of 1 s were used to collect the single-pulse 27 Al MAS NMR spectrum with 240 scans. A pulse width of 0.83 µs corresponding to a π/6 flip-angle and a recycle delay of 2 s were used to collect the single-pulse 17 O MAS NMR spectrum with 1500 scans as well. Note that the small flip-angle single-pulse experiment was used for acquiring 1D 17 O MAS NMR spectra, which is less susceptible to the relatively short recovery delays. In principle, any non-negligible chemical shift anisotropy (CSA) should be considered for quantitative analysis of the 1D 17 O MAS NMR spectrum at high field. To this end, the 17 O NMR spectra (Supplementary Fig. 8 ) were acquired and compared at two different MAS speeds (15 and 40 kHz) with two different relaxation delays (0.5 and 2 s respectively), which reveals that the relaxation and CSA do not have significant influence on our analysis. 2D 1 H { 17 O} J -HMQC spectra of γ-Al 2 O 3 were collected at 18.8 T with a MAS speed of 40 kHz by using a 1.9 m double-resonance probe. A total of 256 scans were collected for each of the 32 rotor-synchronized t 1 increments with a recycle delay of 2 s. 2D 1 H { 17 O} D -HMQC spectra of γ-Al 2 O 3 dehydrated at 473 K were collected using SR4 recouplings with τ re = 1.05 ms and 0.30 ms at a spinning speed of 40 kHz, respectively. A total of 512 scans ( τ re = 1.05 ms) and 128 scans ( τ re = 0.30 ms) were collected for each of the 32 rotor-synchronized t 1 increments with recycle delays of 2 s. 2D 1 H { 17 O} D -HMQC spectrum of γ-Al 2 O 3 dehydrated at 673 K were collected using SR4 recouplings with τ re = 1.05 ms at a spinning speed of 40 kHz. A total of 256 scans were collected for each of the 32 rotor-synchronized t 1 increments with recycle delays of 4 s. Shorter relaxation delays were used in acquiring the 2D experiments for saving whole acquisition time due to the limit magnet time [42] . Pre-saturation pulses and/or satellite saturation pulses were employed to spoil residual longitude magnetizations at the beginning of each scan. For above 2D experiments, presaturation has been applied with a train of 10 π/2 pulses 20 ms apart. The 1 H transverse relaxation (T 2 ) is measured by using a pseudo 2D experiment (chemical shift (CS)-echo) at 18.8 T with a MAS speed of 40 kHz. The T 2 of the 1 H signal from adsorbed water at 4.5 ppm is ca. 0.23 ms, almost half of that (ca. 0.41 ms) of Al-OH species at 1.2 ppm. The chemical shifts were referenced to liquid H 2 O, which is 0 ppm for 17 O and 4.8 ppm for 1 H. Simulations Simulations were performed with the SIMPSON software [56] , and the powder averaging was performed using 320 crystallites following the REPULSION algorithm. C Q values of two coupled oxygen atoms are 2 MHz and 3 MHz, respectively. X-ray powder diffraction (XRD) experiments XRD patterns were recorded on a Panalytical X’ Pert PRO X-ray diffractometer (40 kV, 40 mA) using CuKα ( λ = 1.5406 Å) radiation. The scan rate is 0.05 degrees per second for XRD measurements. TEM measurement TEM image was obtained on a HITACHI HT7700 instrument at an accelerating voltage of 100 kV. IR measurement Diffuse reflectance Fourier transform infrared (DRIFT) spectra were acquired on a Bruker Tensor 27 spectrometer which equipped with CaF2 windows. The samples were packed into the DRIFT cell in a glovebox under dry nitrogen atmosphere. 128 scans were accumulated by a mercury-cadmium telluride (MCT) detector for each spectrum (resolution, 2 cm −1 ), and the background spectrum was collected by KBr.